S-nitrosylation of phosphotransfer proteins represses cytokinin signaling Cytokinin is an essential phytohormone in plant growth and development. In Arabidopsis , cytokinin signalling is mediated by a phosphorelay that sequentially transfers phosphoryl groups from the cytokinin receptors to histidine phosphotransfer proteins (AHPs) and response regulators (ARRs). However, little is known about the regulatory mechanism of the phosphorelay. Here, we show that nitric oxide negatively regulates cytokinin signalling by inhibiting the phosphorelay activity through S -nitrosylation. S -nitrosylation of AHP1 at Cys 115 represses its phosphorylation and subsequent transfer of the phosphoryl group to ARR1. A non-nitrosylatable mutation of AHP1 renders the mutant protein insensitive to nitric oxide in repressing its phosphorylation, and partially relieves the inhibitory effect of nitric oxide on the cytokinin response. Conversely, a nitrosomimetic mutation of AHP1 causes reduced phosphorylation of AHP1 and ARR1, thereby resulting in a compromised cytokinin response. These findings illustrate a mechanism by which redox signalling and cytokinin signalling coordinate plant growth and development. Cytokinin is a key growth-prompting phytohormone that is involved in various aspects of plant growth and development, including in the regulation of root and shoot growth, photomorphogenesis, flowering time, leaf senescence, gametogenesis, embryogenesis and seed development [1] . Genetic and biochemical studies in Arabidopsis have revealed that cytokinin signalling is mediated by a two-component system through a phosphorelay by sequential transferring of phosphoryl groups from the cytokinin receptors to downstream components [1] , [2] , [3] . In Arabidopsis , three histidine kinases (HK), AHK2, AHK3 and AHK4/CRE1/WOL (CYTOKININ RESPONSE 1/WOODEN LEG) have been characterized as the cytokinin receptors [4] , [5] , [6] , [7] , [8] . Upon binding of cytokinin, the cytokinin receptor is activated by autophosphorylation. The phosphoryl group is transferred from the receptor to phosphotransfer proteins (AHPs), which subsequently transfer the phosphoryl group to downstream components, type-A and type-B response regulators (ARRs). Type-B ARRs are a group of MYB-class transcription factors that are activated upon receiving phosphoryl groups and directly regulate the expression of type-A ARR genes and other downstream targets. Type-A ARRs, in turn, negatively regulate the phosphorelay activity, thereby forming a feedback regulatory loop [2] , [3] . Among the three cytokinin receptors, AHK4/CRE1/WOL possesses kinase activity upon binding of cytokinin but exerts phosphatase activity on AHPs in the absence of the cytokinin. Therefore, cytokinin signalling is mediated by a bidirectional phosphorelay that is regulated by the CRE1/WOL/AHK4 receptor [9] and AHP6, a pseudo AHP that acts as a negative regulator of cytokinin signaling [10] . However, it remains unclear whether the phosphorelay activity is regulated by other factors or mechanisms. Cytokinin actively interacts with other phytohormones to regulate plant growth and development. It has been known that the interaction between cytokinin and auxin, another key growth-promoting phytohormone, has an instrumental role in root development [11] , [12] . However, little is known about the interaction of cytokinin with the stress-related signalling molecules such as nitric oxide (NO), which may have an important role in the regulation of plant growth in response to various environmental conditions. NO has a central role in redox signalling and is involved in the regulation of various cellular activities in all living organisms [13] , [14] , [15] . A major bioactivity of NO is in protein S -nitrosylation, a redox-based posttranslational modification mechanism that covalently links an NO group to the reactive cysteine thiol of a protein to form an S -nitrosothiol [16] , [17] , [18] , [19] , [20] . In higher plants, NO has been extensively associated with biotic and abiotic stresses [13] , [14] , [15] , and several S -nitrosylated proteins involved in these processes have been characterized in Arabidopsis [17] , [18] , [19] , [21] , [22] , [23] , [24] , [25] . In addition, NO has also been associated with the auxin and gibberellin responses through various mechanisms. NO enhances the degradation of the auxin transporter PIN1 [26] and the interaction of the auxin receptor with the auxin signalling repressor Aux/IAA [27] . In the gibberellin pathway, NO promotes the accumulation of the gibberellin signalling repressor DELLA [28] . These observations suggest that the NO-modulated phytohormone response is an important adaptation mechanism for the regulation of plant growth. We report here that NO represses cytokinin signalling by inhibiting the phosphorelay activity through S -nitrosylation, revealing a mechanism through which the cytokinin signalling components perceive and integrate a redox signal in the regulation of plant growth and development. NO negatively regulates cytokinin signalling To explore the possible role of NO in cytokinin signalling, we examined the cytokinin response in two Arabidopsis NO-overproducing mutants, nox1 ( NO overproducer1 ) [29] and gsnor1-3 ( S -nitrosoglutathione (GSNO) reductase1) [30] . Cytokinin inhibits the elongation of roots and hypocotyls. When treated with cytokinin, gsnor1-3 and nox1 mutants showed a decreased sensitivity to cytokinin in the inhibition of root and hypocotyl elongation ( Fig. 1a ). The developmental defects and the reduced cytokinin sensitivity of gsnor1-3 were fully rescued by a GSNOR1 - GFP (green fluorescent protein) transgene ( Supplementary Fig. S1 ). However, the overexpression of GSNOR1 did not appear to affect the cytokinin response ( Supplementary Fig. S1c,d ), which is similar to that observed in R gene-mediated resistance and fungi immunity in plants [30] . 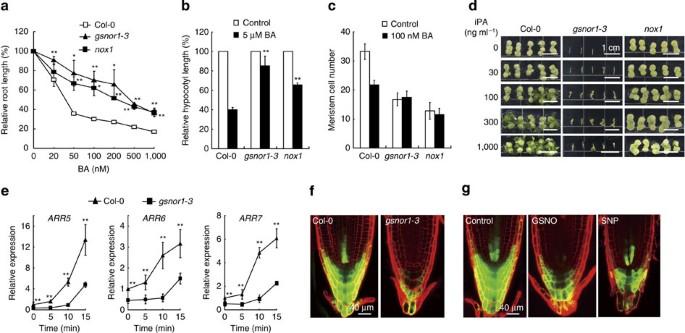Figure 1: Nitric oxide negatively regulates the cytokinin response. (a,b) Analysis of the relative length of the primary roots (a) and hypocotyls (b) of seedlings treated with or without BA. The lengths of roots (a) or hypocotyls (b) not exposed to cytokinin treatment are set at 100% (n≥30) in each genotype. (c) Analysis of the root meristem cell number of seedlings treated with or without BA (n=20). (d) Shoot regeneration capacity of the hypocotyl explants cultured for four weeks in the presence of various concentrations of 2-isopentenyladenine (iPA). (e) Analysis ofARR5,ARR6andARR7expression by qRT–PCR in 10-day-old seedlings treated with 5 μM BA. (f) Confocal microscopy ofTCS-GFPreporter activity in Columbia-0 (Col-0) andgsnor1-3roots. (g)TCS-GFPreporter activity in the roots of 7-day-old Col-0 seedlings grown in the absence (control) or presence of GSNO (400 μM) or sodium nitroprusside (SNP) (100 μM). Error bars indicate s.d.; * and ** indicateP<0.05 andP<0.01, respectively, (Student’st-test). Figure 1: Nitric oxide negatively regulates the cytokinin response. ( a , b ) Analysis of the relative length of the primary roots ( a ) and hypocotyls ( b ) of seedlings treated with or without BA. The lengths of roots ( a ) or hypocotyls ( b ) not exposed to cytokinin treatment are set at 100% ( n ≥30) in each genotype. ( c ) Analysis of the root meristem cell number of seedlings treated with or without BA ( n =20). ( d ) Shoot regeneration capacity of the hypocotyl explants cultured for four weeks in the presence of various concentrations of 2-isopentenyladenine (iPA). ( e ) Analysis of ARR5 , ARR6 and ARR7 expression by qRT–PCR in 10-day-old seedlings treated with 5 μM BA. ( f ) Confocal microscopy of TCS - GFP reporter activity in Columbia-0 (Col-0) and gsnor1-3 roots. ( g ) TCS - GFP reporter activity in the roots of 7-day-old Col-0 seedlings grown in the absence (control) or presence of GSNO (400 μM) or sodium nitroprusside (SNP) (100 μM). Error bars indicate s.d. ; * and ** indicate P <0.05 and P <0.01, respectively, (Student’s t -test). Full size image Cytokinin regulates root meristem size in Arabidopsis [31] . Treatment with cytokinin caused the reduced cortex cell number in the root meristem, and this inhibitory effect was nearly abolished in gsnor1-3 and nox1 ( Fig. 1c and Supplementary Fig. S2 ). Together with auxin, cytokinin specifically promotes shoot regeneration from excised explants, which represents a highly specific assay for the cytokinin response [4] . Cytokinin-induced shoot regeneration from hypocotyl explants was completely lost in gsnor1-3 and significantly reduced in nox1 ( Fig. 1d ). Cytokinin-induced expression of all the tested type-A ARRs , the primary response genes of cytokinin signalling, was substantially reduced in gsnor1-3 ( Fig. 1e and Supplementary Fig. S3 ). Moreover, the expression level and the expression domain of a TCS-GFP cytokinin reporter gene [11] were dramatically reduced in gsnor1-3 roots ( Fig. 1f ). A similar phenotype was also observed in wild-type roots treated with the NO donors GSNO and sodium nitroprusside ( Fig. 1g ). These results demonstrate that NO negatively regulates cytokinin signalling. AHP1 is S -nitrosylated at Cys 115 We reasoned that the downregulation of cytokinin signalling by NO might be caused by S -nitrosylation of key TCS components. In a genome-wide prediction of the putative S -nitrosylated TCS components in Arabidopsis , we identified multiple putative S -nitrosylated cysteine residues in AHKs, AHPs and ARRs, many of which were highly conserved in each class of proteins ( Supplementary Figs S4–S6 ). To test the possible regulatory role of S -nitrosylation in cytokinin signalling, we first examined whether AHPs are S -nitrosylated using the biotin-switch method [32] . S -nitrosylation of His- or GST 4CS - (see Methods and Supplementary Fig. S7 ) tagged AHP1, AHP2, AHP3 and AHP5 recombinant proteins was specifically induced by GSNO and S -nitroso-cysteine (Cys-NO), but not by glutathione (GSH) ( Fig. 2a and Supplementary Fig. S8 ). Similarly, GFP-tagged AHP1, AHP2, AHP3 and AHP5 proteins were S -nitrosylated when transiently expressed in tobacco leaves ( Supplementary Fig. S9 ). 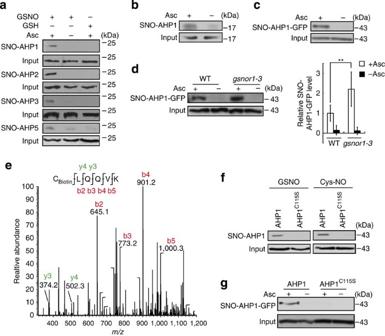Figure 2: AHP1 isS-nitrosylated at Cys 115. (a)S-nitrosylation of recombinant His-tagged AHPs (SNO)in vitro. (b,c)S-nitrosylation of endogenous AHP1 (b) and transgenic AHP1-GFP (c) proteins in Columbia-0 (Col-0) andAHP1::AHP1-GFPseedlings. (d) Accumulation ofS-nitrosylated AHP1-GFP in wild-type (WT) andgsnor1-3plants. A quantitative analysis of the data is shown at the right (n=3). Error bars indicate s.d.; **indicatesP<0.01 (Student’st-test). (e) Mass spectrometric analysis of the tryptic fragments of GSNO-treated GST4CS-AHP1 recombinant protein. The N-terminal fragments (b2 through b5) are charged with biotin, thereby identifying Cys 115 as theS-nitrosylated residue. (f)S-nitrosylation of GST4CS-AHP1 and GST4CS-AHP1C115Srecombinant proteins. (g)S-nitrosylation of AHP1-GFP and AHP1C115S-GFP proteinsin vivo. Figure 2: AHP1 is S -nitrosylated at Cys 115. ( a ) S -nitrosylation of recombinant His-tagged AHPs (SNO) in vitro . ( b , c ) S -nitrosylation of endogenous AHP1 ( b ) and transgenic AHP1-GFP ( c ) proteins in Columbia-0 (Col-0) and AHP1 :: AHP1 - GFP seedlings. ( d ) Accumulation of S -nitrosylated AHP1-GFP in wild-type (WT) and gsnor1-3 plants. A quantitative analysis of the data is shown at the right ( n =3). Error bars indicate s.d. ; **indicates P <0.01 (Student’s t -test). ( e ) Mass spectrometric analysis of the tryptic fragments of GSNO-treated GST 4CS -AHP1 recombinant protein. The N-terminal fragments (b2 through b5) are charged with biotin, thereby identifying Cys 115 as the S -nitrosylated residue. ( f ) S -nitrosylation of GST 4CS -AHP1 and GST 4CS -AHP1 C115S recombinant proteins. ( g ) S -nitrosylation of AHP1-GFP and AHP1 C115S -GFP proteins in vivo . Full size image By the use of an in vivo biotin-switch method [32] (see Methods for details), we found that AHP1 was S -nitrosylated in planta under normal growth conditions ( Fig. 2b ). Similarly, S -nitrosylation of the transgenic AHP1-GFP protein was specifically detected in planta under normal growth conditions ( Fig. 2c ). As GFP-tagged AHP proteins were fully functional ( Supplementary Fig. S10 ), we used the AHP-GFP transgenic plants for most of the experiments described below. Consistently, the accumulation of S -nitrosylated AHP1-GFP was more abundant in gsnor1-3 than in wild-type plants ( Fig. 2d ), which may account for, in part, the altered cytokinin response in gsnor1-3 . Interestingly, treatment with cytokinin induces an increased NO level [33] (see also Supplementary Fig. S11 ), suggesting the possible involvement of a reciprocal regulatory mechanism between the NO and cytokinin signalling pathways. Collectively, these results demonstrate that AHP1 is S -nitrosylated in planta under normal growth conditions. Mass spectrometric analysis of the GSNO-treated AHP1 recombinant protein identified Cys 115 as an S -nitrosylated residue ( Fig. 2e and Supplementary Fig. S12a ). The substitution of Cys 115 with serine abolished the S -nitrosylation of AHP1 both in vitro and in vivo ( Fig. 2f and Supplementary Fig. S12b ). However, S -nitrosylation was not affected in AHP1 C112S -GFP ( Supplementary Fig. S13 ). Consistent with these results, Cys 115 and its flanking sequences in AHP1 partially match the S -nitrosylation consensus motif [16] ( Supplementary Fig. S5a ), and Cys 115 is surrounded by Phe 103 and Arg 114 ( Supplementary Fig. S5b ), a typical acid-base/hydrophobic motif proposed for S -nitrosylation [16] . These results demonstrate that Cys 115 of AHP1 is specifically S -nitrosylated in vivo . S -nitrosylation of AHP1 represses phosphorylation S -nitrosylation regulates the activity of a protein by distinctive mechanisms, including its stability, subcellular localization and biochemical activity [16] , [17] , [18] . We found that mutations at Cys 115 did not affect the subcellular localization or stability of AHP1-GFP ( Supplementary Figs S14,S15 ). Moreover, the gsnor1-3 and nox1 mutations did not have substantial effects on the subcellular localization and stability of AHP proteins ( Supplementary Figs S16,S17 ). We then assessed the phosphorylation of AHP1 and its mutant proteins using a phosphotransfer assay. In this assay, the HK domain and the receiver domain (REC) of the yeast SLN1 HK, a functional ortholog of the cytokinin receptor AHK4/CRE1/WOL [4] , were incubated with wild-type or mutant AHP1 proteins in the presence of 32 γ-ATP, and the sequential transfer of the phosphoryl group through these components was examined by monitoring the radioactivity [9] , [10] . Treatment with GSNO caused a reduction in the transfer of the phosphoryl group from SLN1-REC to AHP1 in a dose-dependent manner ( Fig. 3a ). However, AHP1 C115S , a non-nitrosylatable mutant, was nearly insensitive to GSNO in the phosphotransfer assay ( Fig. 3b ). Conversely, AHP1 C115W , a mutant mimicking S -nitrosylation modification [34] , [35] , [36] , showed the reduced transfer of the phosphoryl group from SLN1-REC to AHP1 C115W ( Fig. 3c ), a phenotype remarkably similar to that of GSNO-treated AHP1. Notably, when a reduced level of SLN1-REC was used in the assay, a decreased phosphorylation level was also observed in GSNO-treated AHP1 and AHP1 C115W , whereas a significantly higher level of radioactivity was retained in the SLN1-REC fraction ( Supplementary Fig. S18 ). Moreover, the transfer of the phosphoryl group to ARR1, a component acting downstream of AHPs during phosphorelay, was substantially reduced when incubated with GSNO-treated AHP1 ( Fig. 4a ) and AHP1 C115W ( Fig. 4b ). These results indicate that S -nitrosylation of AHP1 at Cys 115 represses overall phosphorylation activity during cytokinin-mediated phosphorelay. 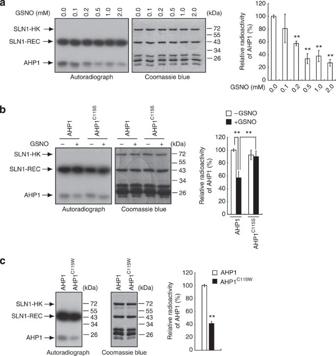Figure 3:S-nitrosylation at Cys 115 causes reduced phosphorylation of AHP1. (a) Inhibition of the phosphorylation of His-AHP1 by GSNO. (b) Effects of GSNO on the phosphorylation of His-AHP1 and His-AHP1C115Srecombinant proteins. (c) The phosphorylation of His-AHP1 and His-AHP1C115Wrecombinant proteins. Quantitative analysis of the relative radioactivity of the target bands is shown on the right side of each panel, and the relative radioactivity of untreated His-AHP1 is set at 100%. All data are presented as mean values of three independent experiments. Error bars indicate s.d.; **indicatesP<0.01 (Student’st-test). Figure 3: S -nitrosylation at Cys 115 causes reduced phosphorylation of AHP1. ( a ) Inhibition of the phosphorylation of His-AHP1 by GSNO. ( b ) Effects of GSNO on the phosphorylation of His-AHP1 and His-AHP1 C115S recombinant proteins. ( c ) The phosphorylation of His-AHP1 and His-AHP1 C115W recombinant proteins. Quantitative analysis of the relative radioactivity of the target bands is shown on the right side of each panel, and the relative radioactivity of untreated His-AHP1 is set at 100%. All data are presented as mean values of three independent experiments. Error bars indicate s.d. ; **indicates P <0.01 (Student’s t -test). 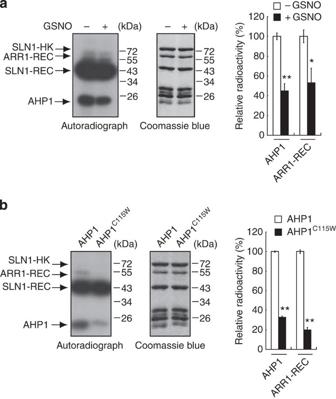Figure 4:S-nitrosylation of AHP1 causes reduced phosphorylation of ARR1. (a) Effects of GSNO on the phosphorylation of MBP-ARR1-REC. (b) Effects of the AHP1C115Wmutation on the phosphorylation of MBP-ARR1-REC. Quantitative analysis of the relative radioactivity of the target bands is shown on the right side of each panel, and the relative radioactivity of untreated MBP-ARR1-REC is set at 100%. All data are presented as mean values of three independent experiments. Error bars indicate s.d.; * and ** indicateP<0.05 andP<0.01, respectively (Student’st-test). Full size image Figure 4: S -nitrosylation of AHP1 causes reduced phosphorylation of ARR1. ( a ) Effects of GSNO on the phosphorylation of MBP-ARR1-REC. ( b ) Effects of the AHP1 C115W mutation on the phosphorylation of MBP-ARR1-REC. Quantitative analysis of the relative radioactivity of the target bands is shown on the right side of each panel, and the relative radioactivity of untreated MBP-ARR1-REC is set at 100%. All data are presented as mean values of three independent experiments. Error bars indicate s.d. ; * and ** indicate P <0.05 and P <0.01, respectively (Student’s t -test). Full size image S -nitrosylation of AHP1 causes compromised cytokinin signalling To assess the physiological relevance of S -nitrosylated AHP1, the AHP1 :: AHP1-GFP , AHP1 :: AHP1 C115S -GFP and AHP1 :: AHP1 C115W -GFP transgenes were introduced into the ahp1 , 2-1 , 3 and ahp1 , 2-1 , 3 , 4 , 5 mutants [37] , and the cytokinin responses of these transgenic plants were analysed. Analysis of root elongation and hypocotyl elongation showed that the cytokinin-insensitivity phenotype of ahp1 , 2-1 , 3 and ahp1 , 2-1 , 3 , 4 , 5 was fully rescued by AHP1-GFP and AHP1 C115S -GFP , but not by AHP1 C115W -GFP ( Fig. 5a and Supplementary Fig. S15 ). In a shoot formation assay, AHP1-GFP and AHP1 C115S -GFP , but not AHP1 C115W -GFP , fully rescued the cytokinin-insensitive phenotype of the ahp1 , 2-1 , 3 , 4 , 5 mutant ( Fig. 5c ). Root protoxylem differentiation is negatively regulated by cytokinin, and the ahp1 , 2-1 , 3 , 4 , 5 quintuple mutation transforms all vascular cells into protoxylem [37] . Whereas AHP1-GFP and AHP1 C115S -GFP restored the ahp1 , 2-1 , 3 , 4 , 5 mutant phenotype to an ahp2-1 , 3 , 4 , 5 -like phenotype, AHP1 C115W -GFP was incapable of rescuing the ahp1 , 2-1 , 3 , 4 , 5 mutant phenotype ( Fig. 5d ). 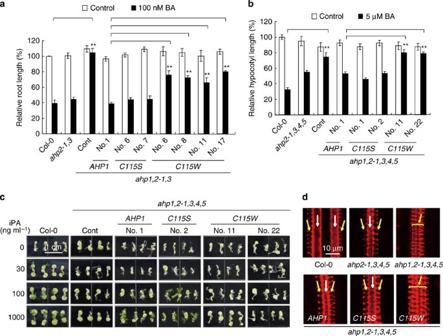Figure 5: Reduced cytokinin response by a nitrosomimetic mutation. (a,b) Analysis of the relative length of roots (a) and hypocotyls (b) in response to the cytokinin BA (numbers refer to the transgenic lines;n≥30). (c) Analysis of the shoot regeneration capacity of hypocotyl explants cultured for 2 weeks in the presence of various concentrations of 2-isopentenyladenine (iPA). (d) Analysis of root xylem development. Protoxylem and metaxylem are indicated by yellow and white arrows, respectively. ‘Cont’ indicates the respective mutants without a transgene in (a–c). All data are presented as mean values of three independent experiments. Error bars indicate s.d.; **indicatesP<0.01 (Student’st-test). Figure 5: Reduced cytokinin response by a nitrosomimetic mutation. ( a , b ) Analysis of the relative length of roots ( a ) and hypocotyls ( b ) in response to the cytokinin BA (numbers refer to the transgenic lines; n ≥30). ( c ) Analysis of the shoot regeneration capacity of hypocotyl explants cultured for 2 weeks in the presence of various concentrations of 2-isopentenyladenine (iPA). ( d ) Analysis of root xylem development. Protoxylem and metaxylem are indicated by yellow and white arrows, respectively. ‘Cont’ indicates the respective mutants without a transgene in ( a – c ). All data are presented as mean values of three independent experiments. Error bars indicate s.d. ; **indicates P <0.01 (Student’s t -test). Full size image Treatment with GSNO attenuated the cytokinin response of the wild-type and AHP1-GFP transgenic plants (in the ahp1 , 2-1 , 3 mutant background) in a root elongation assay ( Fig. 6a ), a phenotype similar to that observed in gsnor1-3 and nox1 that had the elevated levels of NO (see Fig. 1a ). However, the AHP1 C115S -GFP transgenic seedlings displayed the significantly decreased sensitivity to GSNO in the cytokinin-inhibited root elongation ( Fig. 6a ). Cytokinin caused the reduced cell number of the root meristem, and this response is remarkably decreased in the ahp1 , 2-1 , 3 mutant. This cytokinin-insensitive phenotype was rescued by AHP1-GFP and AHP1 C115S -GFP , but not by AHP1 C115W -GFP ( Fig. 6b , left side). Similarly, in root meristem development, GSNO-induced reduction in cytokinin sensitivity was substantially relieved by the AHP1 C115S -GFP transgene ( Fig. 6b , right side). Therefore, the reduced GSNO sensitivity of the AHP1 C115S -GFP transgenic phenotype was consistent with the observation that the AHP1 C115S protein exhibited a reduced response to the inhibitory effect of GSNO on its phosphorylation (see Fig. 3b ). Notably, the AHP1 C115W -GFP transgenic plants showed a ahp1 , 2-1 , 3 -like phenotype in the absence or presence of GSNO ( Fig. 6 ). Taken together, these results indicate that the S -nitrosylation at Cys 115 of AHP1, but not a mutation-induced conformational change, causes a compromised cytokinin response. 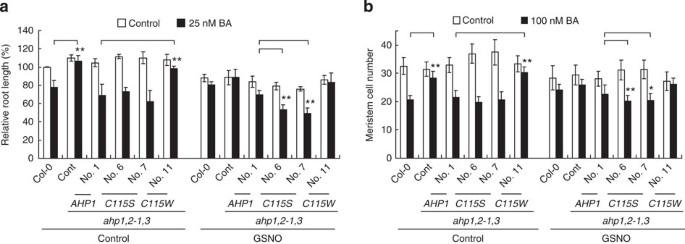Figure 6:S-nitrosylation of AHP1 causes compromised cytokinin signalling. (a,b) Analysis of the relative root length (a) and the root meristem cell number (b) of seedlings treated with various combinations of GSNO (100 μM) and BA (n≥20 in each experiment). All data are presented as mean values of three independent experiments. ‘Cont’ indicates the respective mutants without a transgene. Error bars indicate s.d.; * and ** indicateP<0.05 andP<0.01, respectively, (Student’st-test). Figure 6: S -nitrosylation of AHP1 causes compromised cytokinin signalling. ( a , b ) Analysis of the relative root length ( a ) and the root meristem cell number ( b ) of seedlings treated with various combinations of GSNO (100 μM) and BA ( n ≥20 in each experiment). All data are presented as mean values of three independent experiments. ‘Cont’ indicates the respective mutants without a transgene. Error bars indicate s.d. ; * and ** indicate P <0.05 and P <0.01, respectively, (Student’s t -test). Full size image As a common strategy to cope with stresses and environmental alterations, plants usually respond by regulating the growth rate, which is executed in part by modulating signalling of growth-promoting regulators. The discovery that the S -nitrosylation of AHP1 represses its phosphorylation and consequently attenuates cytokinin signalling, uncovers a molecular mechanism for the perception of a redox signal by the cytokinin signalling components, thereby coordinating plant growth and development. Moreover, the presence of multiple putative S -nitrosylated cysteine residues in AHKs and ARRs implies the involvement of a complex regulatory mechanism, which may be mechanistically different from the regulatory mechanisms that are based on NO synthase-like activity [33] , [38] . In addition, cytokinin induces the production of NO, and mutations in the TCS signalling components impair this response [33] . We speculate that the cytokinin-induced NO burst may act to deactivate cytokinin signalling through S -nitrosylation, thereby establishing a negative feedback loop between NO and cytokinin signalling. The responses of several other growth-promoting phytohormones have been found to be regulated by the cellular redox status. Although the thiol reduction pathways have important roles in the regulation of auxin metabolism and transport [39] , the pleiotropic phenotype of nox1 and gsnor1-3 has been associated with abnormal auxin and gibberellin responses through the regulation of key signalling components in these pathways [26] , [27] , [28] . NO induces the degradation of the auxin transporter PIN1 [26] and stabilizes the gibberellin signalling repressor DELLA [28] , suggesting that NO negatively regulates the responses of auxin and gibberellin, possibly in a similar manner as observed in the NO-repressed cytokinin signalling. Notably, NO has been found to promote auxin signalling by S -nitrosylation of the auxin receptor TIR1, and this modification enhances the interaction between TIR1 and AUX/IAA, thereby facilitating the degradation of AUX/IAA [27] . Moreover, NO stimulates auxin-mediated cell division and embryogenic cell formation in leaf protoplasts of alfalfa [40] . These observations suggest that NO has important roles in the regulation of the auxin and gibberellin responses at multiple levels through distinctive mechanisms, which may repress or enhance specific phytohormone signalling depending on specific environmental conditions and/or developmental stages. Therefore, the NO-modulated signalling of growth-promoting phytohormones is likely to be a general regulatory mechanism, through which plants adjust and adapt their growth in response to dynamic changes of various internal and environmental cues. S -nitrosylation may also regulate the TCS components in response to an NO signal in other organisms. In Salmonella , the response regulator SsrB, a key component of the TCS, is S -nitrosylated upon induction by nitrosative stress, which enhances the fitness against NO produced during the host immune response [41] . The TCS itself, in turn, also has an important role in the adaptation of nitrosative stresses in bacteria [41] , [42] , [43] . Therefore, the S -nitrosylation of TCS components appears to be an evolutionarily conserved mechanism that regulates distinctive physiological activities. Plant materials and growth conditions The Arabidopsis wild-type accession Columbia-0 (Col-0) and related mutants were used in this study. The gsnor1-3 [30] , nox1 [29] and ahp multiple [37] mutant seeds were provided by G. Loake, Z. Pei/Y. He and J. Kieber, respectively. The TCS-GFP reporter line and the TCS-GFP reporter gene [11] were provided by B. Müller and J. Sheen. The TCS-GFP/ gsnor1-3 line was generated by crossing the TCS-GFP reporter line with the gsnor1-3 mutant. The AHP :: AHP - GFP / gsnor1-3 lines were constructed by transformation of heterozygous gsnor1-3 plants with AHP :: AHP - GFP constructs. Seeds were germinated on half-strength MS agar plates containing 1% sucrose. The plates were imbibed at 4 °C for 3 days and then cultured at 22 °C under continuous white light. Transgenic Arabidopsis plants were generated via Agrobacterium -mediated transformation [44] . For all transgenic studies, 4–8 independent transgenic lines were analysed, and similar results were obtained. Representative results were presented. The GV3101 strain of Agrobacterium tumefaciens was used in all genetic transformation experiments in Arabidopsis and tobacco ( Nicotiana benthamiana ). In the tobacco leaf transformation experiments, A . tumefaciens strain GV3101 cells carrying various constructs were mixed with p19 strain before infiltration, and the infiltration was performed by depressing the plunger of a syringe to the surface of leaves [45] . Plasmid construction The GST protein is S -nitrosylated [16] . To prepare GST fusion proteins for S -nitrosylation analysis, we first constructed a modified expression vector. To eliminate the S -nitrosylation sites, we mutated all four cysteines of GST to serines in a pGEX4T-1 vector (Amersham Biosciences) to yield pGST 4CS . Compared with wild-type GST, the GST 4CS mutant protein does not have detectable effects on the expression of the tested target genes, and S -nitrosylation is completely eliminated ( Supplementary Fig. S7 ). The coding sequences of AHP1 , AHP2 , AHP3 and AHP5 were PCR-amplified from Arabidopsis cDNA, and the stop codons were eliminated. These genes were then cloned into the BamH I and Sal I sites of pGST 4CS and pET28a (Novagen) to generate pGST 4CS -AHP and pHis-AHP expression vectors, respectively. The coding sequence corresponding to the REC of ARR1 was amplified from Arabidopsis cDNA and cloned into the BamH I and Sal I sites of pMAL-c2x (New England Biolabs) to generate the pMBP-ARR1-REC expression vector. The coding sequences corresponding to the HK domain and REC of SLN1 were amplified from the genomic DNA of S . cerevisiae and cloned into the BamH I and Sal I sites of pGST 4CS to yield pGST 4CS -SLN1-HK and pGST 4CS -SLN1-REC, respectively. A genomic fragment of GSNOR1 that includes the putative promoter sequence and the coding region was amplified by PCR using wild-type Arabidopsis genomic DNA as a template. The stop codon of GSNOR1 was eliminated, and the appropriate restriction sites were introduced during PCR. The PCR fragment was digested with Xho I/ Sma I and cloned into the Xho I and Sma I sites of pSK-GFP to generate pSK-GSNOR1::GSNOR1-GFP, which was released by Xho I and Xba I and cloned into the Xho I/ Spe I sites of the binary vector pER8 [46] . To create the pSK-AHP::AHP-GFP constructs, genomic fragments of AHP s that include the putative promoter sequences and the coding regions were amplified by PCR using wild-type Arabidopsis genomic DNA as a template. In these PCR fragments, the stop codons were eliminated and the appropriate restriction sites were introduced during PCR. The PCR fragments were digested with Sma I and cloned into the Sma I site of a pSK-GFP vector to generate AHP :: AHP - GFP fusion genes. The 3′-untranslated regions of AHP2 , AHP3 and AHP5 obtained by PCR were inserted downstream of the respective AHP - GFP genes using the BamH I and Spe I sites in the vector. These fusion genes were released by Xho I and Spe I digestion and cloned into the Xho I and Spe I sites of the binary vector pER8 [46] . To construct 35S:: AHP-GFP expression vectors, the coding sequences of each AHP gene were amplified using reverse-transcribed Arabidopsis cDNA as a template and were then fused in-frame to GFP in the pSK-GFP vector using a similar approach as described above. The AHP-GFP fusion genes were subsequently cloned into the Kpn I and Xba I sites of pWM101 under the control of a double 35S promoter [47] . Site-directed mutagenesis was performed using the Easy Mutagenesis System (TransGen Biotech, Beijing) according the manufacturer’s instructions. All PCR-amplified fragments in the constructs described above were confirmed by DNA sequencing analysis, and all constructs were verified by extensive restriction digests. All PCR primers used in this study are listed in Supplementary Table S1 . Quantitative reverse transcription PCR (qRT–PCR) Total RNA was isolated with the RNeasy Plant Mini Kit (Qiagen). Real-time PCR was performed using the UltraSYBR Mixture (CWBIO) according to the manufacturer’s instructions. The reactions were run in a CFX96 REAL-Time PCR Detection System (Bio-Rad). The relative expression level of the target genes was analysed with the delta-delta Ct method and normalized to the expression level of ACTIN7 (At5g09810). All of the experiments were repeated for twice (two biological repeats with 2–3 technical repeats for each experiment) with similar results. Analysis of cytokinin responses To analyse primary root growth, seedlings were grown vertically on agar plates with or without various concentrations of benzyladenine (BA), and root length was measured 7 days post-germination. To measure hypocotyl growth, etiolated seedlings were grown vertically on agar plates containing the appropriate concentrations of BA for 7 days in the dark. To analyse the root meristem size, roots of 7-day-old seedlings were stained with propidium iodide, visualized under a confocal microscope. In the shoot regeneration assay, excised hypocotyls were cultured on the germination medium (full-strength MS salts, 0.05% MES, 1% sucrose, pH 5.8) supplemented with 2,4-D and kinetin for 7 days to induce callus formation, and the calli were transferred onto the germination medium supplemented with indoleacetic acid and different concentrations of 2-isopentenyladenine for 2–4 weeks [48] . The root vasculatures of 7-day-old seedlings were analysed by basic fuchsin red staining [10] and then visualized under a confocal microscope. In planta imaging of NO Analysis of NO contents in roots was performed by DAF-FM diacetate staining (Invitrogen, Cat no. : D23842). Five-day-old seedlings were incubated with various combinations of trans -zeatin ( t ZT; 5 μM) and NO scavenger 2-(4-carboxyphenyl)-4,4,5,5-tetramethylimidazoline-1-oxyl-3-oxide (cPTIO; 1 mM) for 1 h and stained by DAF-FM diacetate for 30 min in the dark. Fluorescence was visualized under a confocal microscope. Expression and purification of recombinant proteins The pMAL- (MBP tag), pET28a- (6XHis tag) and pGST 4CS -based expression vectors were transformed into E . coli BL21. Recombinant proteins were purified using amylose resin (New England Biolabs, Cat no. : E8021S; for the MBP-tagged proteins), 3S-NTA resin (Biocolor Bioscience and Technology Company, Shanghai; for the His-tagged samples) or glutathione Sepharose 4B (GE Healthcare; for the GST 4CS -tagged proteins) following the manufacturers’ instructions. Purified proteins were exchanged for HEN buffer (250 mM Hepes, pH 7.7, 1 mM EDTA) containing 10% (v/v) glycerol or phosphotransfer buffer (50 mM Tris–HCl, pH 7.5, 50 mM KCl, 10% (v/v) glycerol) with Pierce Desalting Cartridges (Pierce Biotechnology, Rockford, IL, USA) following the manufacturer’s instructions. In vivo S -nitrosylation analysis S -nitrosylated proteins were analysed by the biotin-switch assay [32] . Briefly, ~1 g of fresh or frozen samples was homogenized in 1–2 ml of ice-cold HEN buffer (250 mM Hepes, pH 7.7, 1 mM EDTA) containing 0.1 mM neocuproine and protease inhibitor cocktail (Sigma-Aldrich, Cat no. : P9599). The protein extracts were cleared by two rounds of centrifugation at 13,000 g for 10 min at 4 °C. The supernatant was collected, and the concentrated protein extract was diluted to 1 mg ml −1 with HEN buffer. Approximately 100–200 μl of the sample was blocked using blocking buffer 1 (250 mM Hepes, pH 7.7, 1 mM EDTA, 0.1 mM neocuproine, 2.5% SDS, 25 mM S -methylmethane thiosulfonate), and incubated at 50 °C for 30 min with frequent vortexing. The sample was precipitated by adding two volumes of acetone. The pellet was washed three times with 70% acetone and dissolved in 170 μl of HENS buffer (HEN buffer supplemented with 1% SDS) before the addition of 10 μl of 1 M sodium ascorbate and 20 μl of 4 mM biotin-HPDP. After labelling for 90 min at room temperature, the proteins were precipitated with two volumes of acetone. The pellet was briefly washed three times with 50% acetone, dissolved in 400 μl of 250 mM Hepes (pH 7.7), 1 mM EDTA and 1% SDS and neutralized with 800 μl of neutralization buffer (25 mM Hepes, pH 7.7, 100 mM NaCl, 1 mM EDTA, 0.5% Triton X-100). The sample was then mixed with 30 μl of streptavidin beads (Thermo, Cat no. : 29202) and incubated at 4 °C overnight. All of the above manipulations were performed in a dark room with occasional dim light. After the incubation, the beads were washed four times with washing buffer (25 mM Hepes, pH 7.7, 600 mM NaCl, 1 mM EDTA, 0.5% Triton X-100). The proteins were then eluted by boiling in 20 μl of HEN buffer containing 1% 2-mercaptoethanol. The samples were analysed by SDS–PAGE and immunoblotting with the appropriate antibodies, and the blot was quantified using NIH ImageJ (version 1.42q; http://rsbweb.nih.gov/ij/ ). All of the experiments were repeated at least three times with similar results. In vitro S -nitrosylation assay Cys-NO was chemically synthesized [49] . Briefly, equal volume of 200 mM L -cysteine (fresh prepared in 1 M HCl) and 200 mM NaNO 2 (fresh prepared in water) were mixed and then incubated at room temperature in the dark for 30 min, and the reaction was neutralized by adding two volumes of 1 M potassium phosphate (pH 7.4), and stored at −80 °C in small aliquots. Approximately 0.5–2.0 μg of purified recombinant protein was incubated with 100 μM GSNO (Sigma-Aldrich, Cat no. : N4148), Cys-NO or GSH at room temperature in the dark for 10 min (for GST 4CS fusion proteins) or 60 min (for 6 × His fusion proteins), and protein was precipitated by adding three volumes of acetone. The sample was blocked as described above and dissolved in 30 μl of HENS buffer, followed by adding 10 μl of 50 mM sodium ascorbate and 10 μl of 4 mM biotin-HPDP. After labelling for 1 h at room temperature, the sample was directly separated by SDS–PAGE without boiling and analysed by immunoblotting using an anti-biotin antibody (Cell Signalling Technology, Cat no. : 7075). Protein extracts were prepared from Agrobacterium -infiltrated N . benthamiana leaves by homogenization in HEN buffer containing 0.1 mM neocuproine and a protease inhibitor cocktail (Sigma-Aldrich, Cat no. : P9599). The protein concentration of the supernatant was diluted to 1 mg ml −1 with HEN buffer before exposure to 100 μM GSNO for 30–60 min at room temperature in the dark. The biotin-switch assay was then performed as described above. All the experiments were repeated at least three times with similar results. Generation of antibodies and immunoblotting Purified GST-AHP1, GST-AHP2 and 6 × His-AHP3 recombinant proteins were used to immunize rabbits (GST-AHP1 and GST-AHP2) or mice (6 × His-AHP3). The resulting antisera were used directly for immunoblotting. Cytosolic GAPDH served as a loading control using a GAPC antibody [50] (kindly provided by MingChe Shih). The generation and characterization of the anti-GSNOR1 antibody (anti-PAR2 antibody) was described previously [51] . To prepare total cellular proteins, plant materials were grinded in liquid nitrogen, and then extracted in grinding buffer (50 mM Tris-HCl, 150 mM NaCl, 1% Nonidet P-40 and 0.25% sodium deoxycholate) containing protease inhibitor cocktail (Sigma-Aldrich, Cat no. : P9599). After centrifugation twice at 4 °C for 10 min in a microcentrifuge, the supernatant was collected and then subjected to SDS–PAGE. After the run, the proteins were electrically transferred onto a PVDF membrane, and then detected with appropriate antiserum as a primary antibody. The blot was incubated with a secondary antibody (HRP-conjugated goat anti-rabbit IgG or HRP-conjugated goat anti-mouse IgG; Beijing Dingguo Changsheng Biotechnology), and the signal was detected using a SuperSignal Western Femto Maximun Sensitivity Substrate kit (Thermo Scientific, Cat no. : 34096) according to the manufacture’s instructions. Mass spectrometry Approximately 100 μg purified GST 4CS -AHP1 or GST 4CS -AHP1 C115S recombinant proteins were treated with 100 μM GSNO for 1 h in the dark. Excess GSNO was removed by acetone precipitation. The pellet was washed three times with cold acetone, resuspended in blocking buffer 2 (250 mM Hepes, pH 7.7, 1 mM EDTA, 2.5% SDS, 150 mM iodoacetamide) and incubated at 37 °C for 2 h with frequent vortexing. Excess iodoacetamide was removed by acetone precipitation. The pellet was washed three times with acetone and dissolved in HENS buffer containing 50 mM sodium ascorbate and 0.4 mM biotin-HPDP. After labelling for 2 h at room temperature, the proteins were separated by SDS–PAGE without boiling. The target band was excised, washed twice with water and subsequently washed with 50% acetonitrile/25 mM ammonium bicarbonate until transparent. The gel slices were first dehydrated in 50% acetonitrile for 15 min and then completely dehydrated in 100% acetonitrile. After drying, ~50 μl of 10 ng μl −1 trypsin (Promega, Cat no. : V5280) prepared in 50 mM ammonium bicarbonate was added to the dried gel slice, and the sample was incubated at 37 °C for 16 h. The peptides were subsequently extracted twice with 50 μl of 50% acetonitrile/0.5% formic acid for 1 h at 37 °C. The supernatants were combined, concentrated to 20–30 μl, and stored at −20 °C for subsequent analyses. The trypsin-digested sample was analysed by LC-MS/MS using the BioBasic-18 column (0.18 × 150 mm 2 , Surveyor System, Thermo Inc.) coupled on-line with an ion trap mass spectrometer (LCQ Deca Xp plus, Thermo Finnigan). The instrument was run in the data-dependent mode with cycling between one full MS scan from m / z 400–2000 and MS/MS scans of the five most abundant ions using dynamic exclusion. The normalized collision energy was set to 35% for precursor ion fragmentation. The data from MS and MS/MS were used to search the AHP1 protein sequence using the Bioworks 3.1 SR1 (Sequest) software. The search parameters were set to detect four differential modifications: 57 amu on cysteine (indicating carboxyamidomethylation), 71 amu on cysteine (indicating propionamidation), 428 amu on cysteine (indicating biotinylation) and 16 amu on methionine (indicating oxidation). The peptide matching criteria of a cross correlation score (Xcorr) were 1.9, 2.2 and 3.75 for +1, +2 and +3 charged peptides, respectively. Phosphotransfer assay The GSNO treatment was performed by incubating purified His-AHP1 and His-AHP1 C115S recombinant proteins with various concentrations of GSNO for 1 h. Excess GSNO was removed using Zeba Spin Desalting Columns (Thermo, Cat no. : 89883) that were equilibrated with phosphotransfer buffer (50 mM Tris–HCl, pH 7.5, 50 mM KCl, 10% (v/v) glycerol). The phosphotransfer assay was performed as described previously with minor modifications [9] , [10] . The kinase reaction typically contained the following recombinant proteins: 2 μg of GST 4CS -SLN1-HK, 2 μg of GST 4CS -SLN1-REC and 1 μg of His-AHP1 (or the mutants AHP1 C115S and AHP1 C115W ) with or without 1.5 μg of MBP-ARR1-REC. The reaction was carried out at room temperature for 10 min in phosphotransfer buffer supplemented with 5 mM MnCl 2 and 50 μM γ 32 P-ATP (3,000 Ci mmol −1 ), and terminated by the addition of 5 × SDS loading buffer supplemented with 80 mM EDTA. The sample was the subjected to SDS–PAGE without boiling. The gel was stained with Coomassie blue, destained, dried and exposed to X-ray films (CL XPosure Film) at −80 °C. The radioactivity of each band was quantified using NIH ImageJ (version 1.42q, http://rsbweb.nih.gov/ij/ ). All the experiments were repeated for 3–5 times with similar results. Computational modelling The prediction of putative S -nitrosylated cysteine residues was performed by a manual search [16] combined with the use of GPS-SNO software [52] with the threshold set to ‘high’. Modelling of the 3-D structure of AHP1 was performed online at the SwissModel server ( http://swissmodel.expasy.org ) using maize ZmHP2 (PDB: 1WN0) as a template [53] . Molecular graphics were prepared using PyMOL software ( http://www.pymol.org/ ). How to cite this article: Feng, J. et al . S -nitrosylation of phosphotransfer proteins represses cytokinin signaling. Nat. Commun. 4:1529 doi: 10.1038/ncomms2541 (2013).